Anisotropic two-dimensional electron gas at the LaAlO3/SrTiO3(110) interface The observation of a high-mobility two-dimensional electron gas between two insulating complex oxides, especially LaAlO 3 /SrTiO 3 , has enhanced the potential of oxides for electronics. The occurrence of this conductivity is believed to be driven by polarization discontinuity, leading to an electronic reconstruction. In this scenario, the crystal orientation has an important role and no conductivity would be expected, for example, for the interface between LaAlO 3 and (110)-oriented SrTiO 3 , which should not have a polarization discontinuity. Here we report the observation of unexpected conductivity at the LaAlO 3 /SrTiO 3 interface prepared on (110)-oriented SrTiO 3 , with a LaAlO 3 -layer thickness-dependent metal-insulator transition. Density functional theory calculation reveals that electronic reconstruction, and thus conductivity, is still possible at this (110) interface by considering the energetically favourable (110) interface structure, that is, buckled TiO 2 /LaO, in which the polarization discontinuity is still present. The conductivity was further found to be strongly anisotropic along the different crystallographic directions with potential for anisotropic superconductivity and magnetism, leading to possible new physics and applications. Owing to structural, charge, orbital or spin reconstruction at their interfaces, complex oxide heterostructures have emerged as an avenue for creation of exotic phenomena that are absent in their bulk constituents [1] . One of the most exciting systems of such heterostructures is the interface between two band insulators LaAlO 3 and SrTiO 3 . When these two perovskite type oxides are brought together along the (100) orientation, a highly conducting two-dimensional electron gas (2DEG) emerges at their interface [2] . Further, this interface has also been shown to exhibit various electronic and magnetic phases such as a tunable metal-insulator ground state [3] , two-dimensional superconductivity [4] , [5] , magnetic ground state [6] and an electronic phase separation [7] in which different magnetic phases are present together with the interface conductivity. Most recently, the coexistence of mutually exclusive phenomena, magnetism and superconductivity is also reported [8] , [9] , [10] . Nevertheless, all of these studies were specific only to the interfaces constructed along the (100) crystallographic orientation. The conductivity in crystalline LaAlO 3 /SrTiO 3 (100) interface is mostly interpreted to originate from electronic reconstruction, which is a direct consequence of the polarization discontinuity [11] at the interface between the two oxides. In this case, the ABO 3 perovskite structure of the SrTiO 3 (100) substrate can be considered as stacks of (SrO) 0 and (TiO 2 ) 0 ( Fig. 1a ), whereas for the LaAlO 3 , it consists of charged sheets of (LaO) +1 and (AlO 2 ) −1 , which leads to a polarization discontinuity at the interface between the LaAlO 3 and SrTiO 3 . On the other hand, for the case of LaAlO 3 /SrTiO 3 interfaces prepared on SrTiO 3 (110) substrate ( Fig. 1c ), both the SrTiO 3 and LaAlO 3 can be represented by planar stacks of (ABO) +4 and (O 2 ) −4 layers as proposed in Hwang et al. [12] and Mukunoki et al. [13] which leads to no polarization discontinuity at the interface. Consequently, no conductivity would be expected for such LaAlO 3 /SrTiO 3 (110) interfaces. 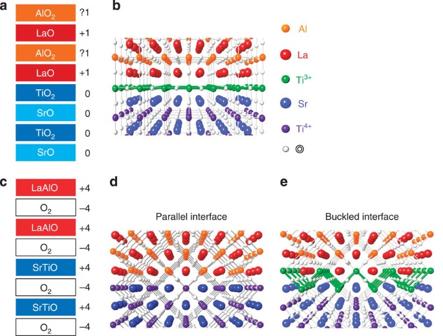Figure 1: Interface configurations. Layout of the polar catastrophe model for LaAlO3/SrTiO3interface on (a) (100)- and (c) (110)-oriented SrTiO3substrates, where planes are segmented as planar charge sheets. In the case of (100), charge transfer is expected, whereas in the case of (110), there is no polarization discontinuity and hence no charge transfer. (b,d) Atomic picture of the interfaces for representations (a) and (c), respectively. (e) Atomic picture of LaAlO3/SrTiO3interface on (110)-oriented SrTiO3, considering the (110) planes of SrTiO3and LaAlO3as buckled sheets. Figure 1: Interface configurations. Layout of the polar catastrophe model for LaAlO 3 /SrTiO 3 interface on ( a ) (100)- and ( c ) (110)-oriented SrTiO 3 substrates, where planes are segmented as planar charge sheets. In the case of (100), charge transfer is expected, whereas in the case of (110), there is no polarization discontinuity and hence no charge transfer. ( b , d ) Atomic picture of the interfaces for representations ( a ) and ( c ), respectively. ( e ) Atomic picture of LaAlO 3 /SrTiO 3 interface on (110)-oriented SrTiO 3 , considering the (110) planes of SrTiO 3 and LaAlO 3 as buckled sheets. Full size image Here we demonstrate that a high-mobility 2DEG can also arise at this LaAlO 3 /SrTiO 3 (110) interface. The (110) interface shows transport property and LaAlO 3 -layer critical thickness for the metal-to-insulator transition similar to those of (100) interfaces, but with a strong anisotropic characteristic along the two in-plane crystallographic directions. This anisotropic behaviour is further found to be sensitive to the oxygen growth condition. The density functional theory (DFT) study shows that the energetically favourable atomic structure along the (110) orientation can support the electronic reconstruction when the interface is represented by an alternate way in which the polarization discontinuity is still present. Electrical transport properties The growth parameters for the LaAlO 3 /SrTiO 3 (110) and (100) samples are discussed in the Methods section. The sheet resistance, R s , charge density, n s , and Hall mobility, μ , were measured using a van der Pauw geometry. 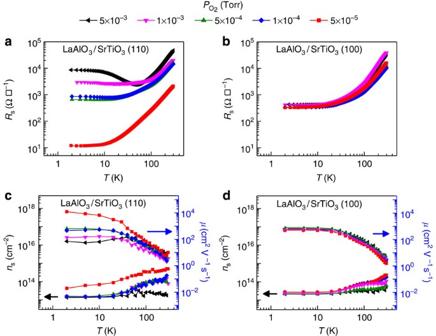Figure 2: Transport properties. Temperature dependence of the sheet resistanceRs(T) of the LaAlO3/SrTiO3interfaces for different oxygen partial pressures () during growth on (a) (110)- and (b) (100)-oriented SrTiO3substrates. Temperature dependence of carrier densityns(T) and Hall mobilityμ(T) of the LaAlO3/SrTiO3interfaces for different during growth on (c) (110)- and (d) (100)-oriented SrTiO3substrates. Figure 2a shows R s versus temperature for the LaAlO 3 /SrTiO 3 (110) samples grown at different oxygen partial pressures ( ) with a fixed thickness of 12 unit-cells (uc) LaAlO 3 . Strikingly, these interfaces show conductivity reminiscent to the (100) case ( Fig. 2b ), albeit with a larger dispersion with respect to the oxygen pressure during growth. The R s follows a T 2 -like dependence over a temperature range of 300–100 K and tends to saturate at low temperatures. The samples grown at higher oxygen pressures show a resistance upturn at lower temperatures, a typical localization/Kondo behaviour indicating the presence of magnetic scattering centres at the interface. Although Kondo scattering in the (100) case is reported only for LaAlO 3 thickness >15 uc (refs 6 , 14 , 15 ), in the case of (110), it is seen even for 10 uc LaAlO 3 thickness, indicating stronger scattering effects. We note here that for the (100) case, the dispersion in the resistivity with oxygen deposition pressures was also reported but for samples with ‘thicker’ LaAlO 3 layers of 20 uc (ref. 6 ), implying different sensitivity to the LaAlO 3 thickness between these interfaces. Interestingly, there is a temperature shift in the resistance-minimum with the oxygen growth pressure, indicating that the strength of the scattering at the interface is sensitive to the deposition conditions. We note here that resistivity measurements have been carried out down to 2 K, and it is feasible that some of these samples may become superconducting at lower temperatures. Figure 2: Transport properties. Temperature dependence of the sheet resistance R s ( T ) of the LaAlO 3 /SrTiO 3 interfaces for different oxygen partial pressures ( ) during growth on ( a ) (110)- and ( b ) (100)-oriented SrTiO 3 substrates. Temperature dependence of carrier density n s ( T ) and Hall mobility μ ( T ) of the LaAlO 3 /SrTiO 3 interfaces for different during growth on ( c ) (110)- and ( d ) (100)-oriented SrTiO 3 substrates. Full size image Figure 2c shows the corresponding variation in n s and μ with temperature for the LaAlO 3 /SrTiO 3 (110) and (100) samples grown at different . For the (110) samples, n s decreases with decreasing temperature, and for the samples grown at higher partial pressures, n s at low temperature (2 K) tends towards a constant value of about 1.5 × 10 13 cm −2 , which is somewhat lower than the residual carrier density of about 2.5 × 10 13 cm −2 for the LaAlO 3 /SrTiO 3 (100) samples. This could be due to the preferred occupancy of the Ti-3d orbitals at the interface, which may localize some of the electrons [16] , [17] . For the thermally activated charge carriers in the (110) samples, we find an activation energy of about 9 meV, whereas in LaAlO 3 /SrTiO 3 (100) interfaces, an activation energy of 6.0 meV has been reported [18] , [19] . For both orientations, the measured μ follows a power law temperature dependence for T >100 K, as μ ~5 × 10 6 T −2.2 . All the samples grown at higher pressures show μ values of the order of 200–600 and 2–7 cm 2 V −1 s −1 at 2 and 300 K, respectively. These values correspond well with those reported in literature for the LaAlO 3 /SrTiO 3 (100) interfaces [3] , [14] , [20] . We notice a decrease in the μ in the (110) case, simultaneous with Kondo features becoming visible in the R s ( T ) curves. For the (110) sample grown at 5 × 10 −5 Torr, the n s at 300 K is 4.9 × 10 14 cm −2 , which has the μ of 12,000 cm 2 V −1 s −1 at 2 K, suggesting contribution from other sources such as oxygen vacancies [20] , [21] and defect centres present near the interface. Thickness-dependent insulator to metal transition One of the characteristic features of the LaAlO 3 /SrTiO 3 (100) interfaces, and considered as one of the most important arguments for a polarization discontinuity driven mechanism, is the dependence of the sheet conductivity on the number of ucs of LaAlO 3 with the observation of an insulator to metal transition at 3–4 uc of LaAlO 3 layers [3] . In Fig. 3 , the conductivity versus the number of LaAlO 3 ucs N grown on the SrTiO 3 (110) substrates is plotted. Here also we clearly see two regimes, an insulating one at low N ( N <3) and a metallic state at higher N ( N ≥4) values. 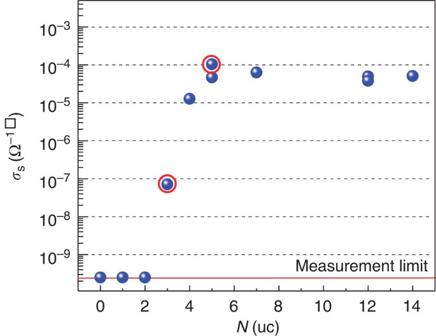Figure 3:LaAlO3thickness dependence of sheet conductivity. The room-temperature sheet conductivity as a function of number of ucs of LaAlO3for the LaAlO3/SrTiO3(110) samples, clearly showing the insulator to metal transition (data points marked with open red circle are for a sample initially having 3 uc of LaAlO3, followed by the growth of two more uc making it 5 uc in total). Figure 3: LaAlO 3 thickness dependence of sheet conductivity. The room-temperature sheet conductivity as a function of number of ucs of LaAlO 3 for the LaAlO 3 /SrTiO 3 (110) samples, clearly showing the insulator to metal transition (data points marked with open red circle are for a sample initially having 3 uc of LaAlO 3 , followed by the growth of two more uc making it 5 uc in total). Full size image Considering all the data presented above, it is remarkable that the (110) samples are not only conducting but also bear remarkable similarities to the conductance properties of the (100) case. However, there are also strong differences, the most noticeable of which is the anisotropy of the conductance. 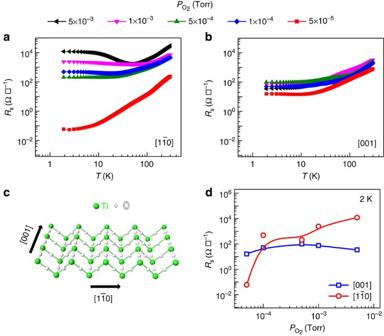Figure 4: Anisotropic conductivity of theLaAlO3/SrTiO3(110) interfaces. Rs(T) measured along (a) [10] and (b) [001] directions for the LaAlO3/SrTiO3(110) samples grown at different oxygen partial pressures. (c) Schematic view of the Ti chain arrangement along the [10] and [001] directions. (d) Deposition oxygen pressure dependence ofRsat 2 K measured along the [10] and [001] directions. Anisotropy of electronic transport Figure 4a show the electrical transport characteristics of the LaAlO 3 /SrTiO 3 (110) samples along the [1 0] and [001] directions, respectively, demonstrating the anisotropic transport behaviour as a function of along the two crystallographic directions. Strikingly, along [1 0] direction, strong localization effects are seen at low temperatures, whereas along [001] direction, such localizations are absent. A basic difference between these two directions is the presence of linear Ti-O-Ti chains along [001] and buckled Ti-O-Ti chains along [1 0] as depicted schematically in Fig. 4c . The deposition pressure dependence of R s at 2 K is plotted in Fig. 4d for both directions. Clearly, the conductivity along the [1 0] direction has a much stronger dependence on deposition pressures compared with the [001] direction, indicating the strong role of the differences in the Ti-O-Ti chain along the two orthogonal directions. The anisotropy arising from other effects such as step edges [22] has been measured for (100) case ( Supplementary Fig. S1 ), and this is substantially smaller than what we see in the (110) case and so we can rule out step edge scattering as the dominant mechanism. Figure 4: Anisotropic conductivity of theLaAlO 3 /SrTiO 3 (110) interfaces. R s ( T ) measured along ( a ) [1 0] and ( b ) [001] directions for the LaAlO 3 /SrTiO 3 (110) samples grown at different oxygen partial pressures. ( c ) Schematic view of the Ti chain arrangement along the [1 0] and [001] directions. ( d ) Deposition oxygen pressure dependence of R s at 2 K measured along the [1 0] and [001] directions. Full size image Origin of conductivity and interface structure The fact that there are many similar properties to the (100) case, even including the insulator to metal transition at around 4 uc of LaAlO 3 , indicates that a very similar mechanism is at work for the formation of the 2DEGs for both (100) and (110) cases. Recently, Stengel et al. [23] discussed the issue of polarity in various oxides, especially the case of LaAlO 3 and SrTiO 3 surfaces, where it is shown that in LaAlO 3 case, the surface with cleavage planes are shown to be energetically favourable than a simple polar (001) surface. In analogous to this, our DFT calculation results suggest that buckled TiO termination at SrTiO 3 (110) surface is more favourable than a hypothetical polar stoichiometric SrTiO surface ( Supplementary Fig. S2 ). In this scenario, the atomic structure of the interface would be critical [23] to determine polarity effects at these heterostructures. We further perform DFT calculations on the LaAlO 3 /SrTiO 3 (110) interface and found that the origin for the unexpected conductivity in the (110) case can also be explained by considering energetically stable buckled TiO termination, resulting in a modified polarization discontinuity with an interface viewed as depicted in Fig. 1e (buckled interface) rather than the one in Fig. 1c (planar interface). The electronic configuration of interfaces with such a buckled interface structure as in Fig. 1e was modelled by DFT as shown in Fig. 5a . Indeed as shown in Fig. 5b , an insulator to metal transition with increasing number of LaAlO 3 monolayers is obtained. The critical thickness for insulator to metal transition is about 4 uc, which is in agreement with our experimental observation. This result shows that by viewing the LaO/TiO 2 as buckled layers, the thickness dependence of the insulator to metal transition arising from avoiding the polarization catastrophe can be reproduced [24] . 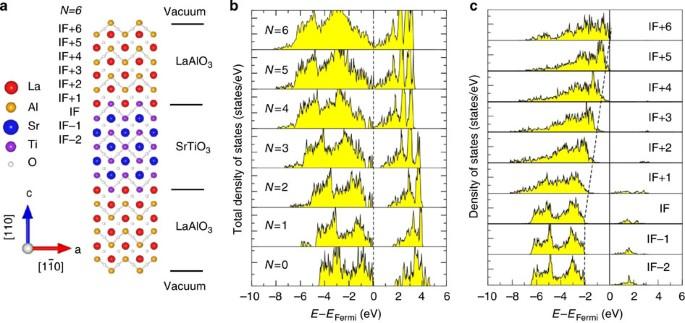Figure 5: DFT calculations. (a) Schematic cell structure of LaAlO3/SrTiO3(110) interface with TiO-terminated SrTiO3(110) for six monolayers of LaAlO3. (b) The total density of states for different numbersNof LaAlO3monolayers deposited on SrTiO3(110) clearly shows the band gap decrease with increasingNand an insulator to metal transition occurring at 4 uc. (c) The partial density of states for O-2p projected onto each layer forN=6 monolayers of LaAlO3deposited onto TiO-terminated (110) SrTiO3. Here the top of valance band for each monolayer is indicated by dashed lines. The Fermi level is denoted byEFermi. Here IF represents interface. Figure 5c shows the partial density of states for O-2p projected onto each layer. From the figure, we can see clearly that the top of the valence band moves towards Fermi level as we approach the surface, suggesting that there can still exists an intrinsic electrostatic fields to avoid the polar catastrophe due to the polar discontinuity caused by the buckled interface. This intrinsic electrostatic field can induce the insulator to metal transition when this electrostatic potential exceeds the band gap. In our case, this transition occurs at N <4 as shown in Fig. 3 . Note, however, the critical value of N might depend on approximations used for calculations; we also find by performing generalized gradient approximation (GGA)+U calculations that the main conclusion are qualitatively the same. Thus, the DFT study reveals that the interface between LaAlO 3 and the energetically favourable atomic structure of the TiO-terminated SrTiO 3 (110) can support the conductivity with the interface that is represented by an alternate way, namely, the buckled interface shown in Fig. 1e , in which the polarization discontinuity is still present. Figure 5: DFT calculations. ( a ) Schematic cell structure of LaAlO 3 /SrTiO 3 (110) interface with TiO-terminated SrTiO 3 (110) for six monolayers of LaAlO 3 . ( b ) The total density of states for different numbers N of LaAlO 3 monolayers deposited on SrTiO 3 (110) clearly shows the band gap decrease with increasing N and an insulator to metal transition occurring at 4 uc. ( c ) The partial density of states for O-2p projected onto each layer for N =6 monolayers of LaAlO 3 deposited onto TiO-terminated (110) SrTiO 3 . Here the top of valance band for each monolayer is indicated by dashed lines. The Fermi level is denoted by E Fermi . Here IF represents interface. Full size image To investigate the possibility of such proposed buckled atomic structure at the (110) interfaces, we performed cross-sectional scanning transmission electron microscopy (STEM) on the LaAlO 3 /SrTiO 3 (110) interfaces. 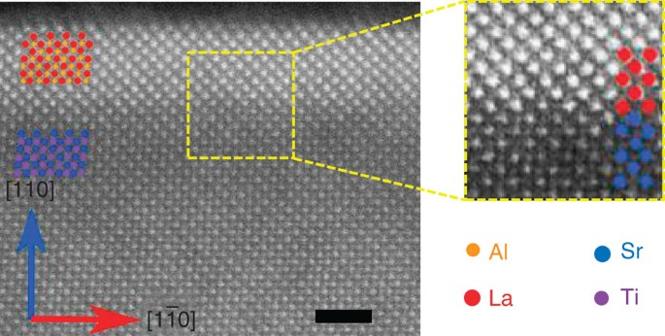Figure 6: Transmission electron microscopy. High-angle annular dark-field STEM images of the LaAlO3film on the SrTiO3(110) substrate shows an epitaxial growth of the LaAlO3/SrTiO3(110) heterostructure (A-site atoms La and Sr are indicated by red and blue, respectively, and theB-site atoms Al and Ti by orange and purple, respectively). A magnified view of the elemental mapping across the interface is also shown on the right side. Scale bar, 2 nm. Figure 6 shows a high-angle annular dark-field STEM image of the LaAlO 3 film grown on the SrTiO 3 (110) substrate. The image shows a perfect epitaxial growth of the LaAlO 3 across the interface of the heterostructure along the (110) orientation. The signal from the atom columns depends on the atomic number [25] . The ratio between the signals of the Al and La atom columns is expected to be <10%. In addition, the projection along the Al atom columns also includes O atoms further adding to the background signal of the Al columns. We also note that the background intensity is generally higher in LaAlO 3 compared with the result of (100) interfaces [26] . The Al and Ti ( B -site) atom columns are visible in the STEM images. However, it is found that it is difficult to use them as indicators of the interface between the LaAlO 3 and SrTiO 3 film on the basis of poor signal to background ratio. Therefore, the La and Sr ( A -site) atom columns have been used as indicators for the film/substrate interface. In Fig. 6 , a higher resolution of elemental mapping at the interface representing the arrangement of La (red) and Sr (blue) positions in both LaAlO 3 and SrTiO 3 is also shown. We notice some of the La and Sr atoms at the interface extend up to 2–4 uc rather than 2 uc as anticipated. Both the sparseness of such extended facets and the absence of connectivity among them rule out other mechanisms for conduction (for example, an effective (100) interface at 45 degrees). However, the models in Fig. 1d cannot be distinguished just by identifying only the A -site cations as in our current STEM data. Therefore, one needs to further resolve the chemical identity of the B -site cations alongside A -site cations to confirm the proposed buckled structure in Fig. 1e . Figure 6: Transmission electron microscopy. High-angle annular dark-field STEM images of the LaAlO 3 film on the SrTiO 3 (110) substrate shows an epitaxial growth of the LaAlO 3 /SrTiO 3 (110) heterostructure ( A -site atoms La and Sr are indicated by red and blue, respectively, and the B -site atoms Al and Ti by orange and purple, respectively). A magnified view of the elemental mapping across the interface is also shown on the right side. Scale bar, 2 nm. Full size image The importance of the (110) interface is better brought out in context with what has been learnt so far with the (100) interfaces. The 2DEG at the LaAlO 3 /SrTiO 3 (100) interfaces has been studied under a variety of deposition conditions, layer thicknesses and externally applied fields [27] , [28] . In most of these experiments, the 2DEG was presumed to be the result of a direct manipulation of electrostatic potential at the interface to promote electrons to the conduction band of SrTiO 3 , which requires energy of the order of 3.2 eV. However, recently the 2DEG was also demonstrated on the surface of SrTiO 3 by shining ultraviolet light [29] , vacuum cleaving [30] and chemical reduction of the surface during growth [31] . It is apparent that the 2DEG can be produced by different mechanisms, which can elevate the electron to the conduction band of SrTiO 3 . Recent experimental work involving amorphous over layers on SrTiO 3 showing a conducting interface has brought in the importance of interface chemistry [31] . Under this scenario, oxygen diffusion from SrTiO 3 surface during film growth into the over layers was deemed responsible for the interface conductivity. What was striking was the similarity of the results between the amorphous and crystalline over layers in terms of the saturation in charge density and conductivity with the film thickness. Unlike their crystalline counterparts, however, one of the short comings of the amorphous over layers seems to be the thermal stability of the interfaces that lose their conductivity subsequent to a 150 °C anneal in air, which will make them unsuitable for device applications (crystalline samples in our case were found to be stable post annealing and preserve conductivity). The real attraction of the crystalline interfaces is that they offer a variety of controllable parameters such as strain [32] , correlation effects [33] through structure coupling and large anisotropy (as shown here), which can be used to manipulate the interface properties. Our experiments and DFT calculations using (110) substrates show that the polarization catastrophe model may still be valid for crystalline LaAlO 3 /SrTiO 3 interfaces, provided the interface is viewed appropriately (buckled interface). Because of the different atomic structure in the (110) interfaces, the presence of buckled Ti-O-Ti chains opens up new possibilities, which may lead to new phenomena. For example, the anisotropy can be further explored by nano-structuring the 2DEG along the anisotropic crystallographic axis with techniques such as charge writing using atomic force microscopy [34] , which is already shown to create new properties. The other effect of the crystallographic anisotropy is on the reported spin-orbit interaction [35] , which would further attract a lot of interest to explore the electric field effects on these anisotropic surfaces. Further investigation of the anisotropy on other phenomena (magnetism and superconductivity) will be of interest for the community and may lead to new physics and device applications. Substrate treatment For the (100) case, substrates were treated with well-established conditions; buffered HF for 30 s followed by thermal annealing at 950 °C for 2 h in air [36] , [37] . For the (110)-oriented SrTiO 3 , the substrates were annealed for 3 h at 1050 °C in air [38] . The step height in this case is about 0.28 nm, which is the uc spacing along the [110] direction. The step edges appear to be facetted along the [001] and [1 0] low-index crystallographic directions, giving rise to the triangular-shaped steps [39] ( Supplementary Fig. S3 ). Reflection high-energy electron diffraction analysis on the SrTiO 3 (110) surface shows a signature of a (1 × 3) reconstructed surface ( Supplementary Fig. S4 ). Sample growth The LaAlO 3 /SrTiO 3 (110) samples were prepared with various LaAlO 3 thicknesses ( N ) from 1 to 14 uc under different ranging from 5 × 10 −5 to 5 × 10 −3 Torr on atomically smooth SrTiO 3 (110) substrates. The LaAlO 3 films were deposited from a single-crystal LaAlO 3 target at 720 °C by pulsed laser deposition. The laser (248 nm) energy density was 1.4 J cm −2 and repetition rate was 1 Hz. During deposition, the film growth was monitored using in-situ reflection high-energy electron diffraction. After deposition, all samples were cooled to room temperature at 10 °C min −1 in oxygen at the deposition pressure. For comparison, LaAlO 3 /SrTiO 3 (100) samples were grown with 12 uc LaAlO 3 layers under the same preparation conditions. Structural analysis Thicker LaAlO 3 films of about 15 nm were grown to enable confirmation of the growth orientation of the LaAlO 3 on SrTiO 3 (110) and (100) substrates by X-ray diffraction ( Supplementary Fig. S5 ). Samples for STEM were prepared by using cutting, mechanical grinding, polishing and low-voltage Ar-ion beam milling as a final polishing step. High-angle annular dark-field STEM images were recorded using a FEI Titan 80–300 microscope with a corrector for spherical aberration of the condenser lenses and a monochromator. The microscope was operated at 300 kV. The electron beam is incident along the [001] direction to the LaAlO 3 /SrTiO 3 (110) interface. Electrical characterization Electrical characteristics for all the samples were measured with the van der Pauw technique. Ohmic contacts onto four corners of a 5 × 5 mm 2 sample were formed using Al wedge bonding directly connected to the sample interface. Sheet carrier density n s and carrier mobility μ were determined as n s =1/ eR H and μ = R H / R s , where R s is the sheet resistance and R H is Hall coefficient. For the directional-dependence transport measurements, crystallographic directions on the surface of substrate were identified as specified by the substrate supplier (Crystec GmbH). Density functional theory First-principles calculations based on the DFT for LaAlO 3 /SrTiO 3 (110) interface was performed. We used the GGA (ref. 40 ) and the projected augmented wave method with a plane wave basis set as implemented in the Vienna Ab initio Simulation Package [41] , [42] , [43] . To study the thickness dependence of LaAlO 3 monolayers deposited on SrTiO 3 (110) substrate, we use a slab model shown in Fig. 5a . Here, as usual, the inversion symmetry of the slab is assumed to avoid spurious electronic field. In all calculations, a vacuum region of 12 Å between repeated slabs is taken. A kinetic energy cut off is set to be 400 eV for the plane wave basis and the slab is sampled with 8 × 8 × 1 k-point grid in combination with the tetrahedron method. Although the in-plane lattice constant is fixed at the relaxed lattice constant of bulk SrTiO 3 ( a =3.944 Å), all coordinates of atomic positions along the c -direction perpendicular to the interface are fully relaxed until the forces become <0.01 eV Å −1 . We have carefully checked the convergence of our calculations. Our calculations show that the energy gap for bulk SrTiO 3 is about 1.8 eV, separating the valence band with O-2p characters and the conduction band mainly composed of Ti-3d. For LaAlO 3 , we obtain the band gap of 3.2 eV. These estimated values of the band gap are similar to the ones previously reported by DFT calculations [34] and are smaller than the ones observed experimentally. However, the underestimation of the energy gap within GGA is well known, and the GGA+U approach, for instance, gives an improved description. How to cite this article: Annadi, A. et al. Anisotropic two-dimensional electron gas at the LaAlO 3 /SrTiO 3 (110) interface. Nat. Commun. 4:1838 doi: 10.1038/ncomms2804 (2013).